The nature of domain walls in ultrathin ferromagnets revealed by scanning nanomagnetometry The capacity to propagate magnetic domain walls with spin-polarized currents underpins several schemes for information storage and processing using spintronic devices. A key question involves the internal structure of the domain walls, which governs their response to certain current-driven torques such as the spin Hall effect. Here we show that magnetic microscopy based on a single nitrogen-vacancy defect in diamond can provide a direct determination of the internal wall structure in ultrathin ferromagnetic films under ambient conditions. We find pure Bloch walls in Ta/CoFeB(1 nm)/MgO, while left-handed Néel walls are observed in Pt/Co(0.6 nm)/AlO x . The latter indicates the presence of a sizable interfacial Dzyaloshinskii–Moriya interaction, which has strong bearing on the feasibility of exploiting novel chiral states such as skyrmions for information technologies. The recent observation of current-induced domain wall (DW) motion with large velocity in ultrathin (few atomic layers) magnetic wires has opened new opportunities for spintronic devices [1] . However, there is still no consensus on the underlying mechanisms of DW motion, and several distinct models have been shown to be consistent with experimental observations [1] , [2] , [3] , [4] , [5] , [6] , [7] . The key to this debate is the DW structure, which can be of Bloch or Néel type, and which dramatically affects the efficiency of the different proposed mechanisms [7] , [8] , [9] . In a wide ultrathin ferromagnetic wire with perpendicular magnetic anisotropy, magnetostatics predicts that the Bloch DW, a helical rotation of the magnetization, is the most stable DW configuration because it minimizes volume magnetic charges [10] . However, the unexpectedly large current-induced DW velocities, recently observed in ultrathin ferromagnets [1] , added to the fact that the motion can be found against the electron flow [2] , [3] , has cast doubt on this hypothesis and triggered a major academic debate regarding the physical processes at the origin of DW motion [4] , [5] , [6] , [7] , [8] , [9] . Notably, it was recently proposed that Néel DWs with fixed chirality could be stabilized by the Dzyaloshinskii–Moriya interaction (DMI) [8] , an indirect exchange possibly occurring at the interface between a magnetic layer and a heavy metal substrate with large spin-orbit coupling [11] . For such chiral DWs, hereafter termed Dzyaloshinskii DWs, a damping-like torque due to spin-orbit terms (spin Hall effect and Rashba interaction) would lead to efficient current-induced DW motion along a direction fixed by chirality [8] . In order to validate unambiguously these theoretical predictions, a direct, in situ , determination of the DW structure in ultrathin ferromagnets is required. However, the relatively small number of spins at the wall centre makes direct imaging of its inner structure a very challenging task. So far, only spin-polarized scanning tunnelling microscopy [12] and spin-polarized low-energy electron microscopy [13] have allowed a direct determination of the DW structure, demonstrating homochiral Néel DWs in Fe double layer on W(110) and in (Co/Ni) n multilayers on Pt or Ir, respectively. However, these techniques are intrinsically limited to model samples because of high experimental constraints, for example bare magnetic surface hence ultrahigh vacuum, and the debate remains open for widely used trilayer systems with perpendicular magnetic anisotropy such as Pt/Co/AlO x (ref. 1 ), Pt/Co/Pt (ref. 4 ) or Ta/CoFeB/MgO (ref. 14 ). Indeed, most experiments aiming to deduce the DW structure and chirality in such trilayer systems have relied on DW motion analysis under additional in-plane applied fields, which is indirect and involves strong assumptions on the DW dynamics [2] , [3] , [4] , [14] , [15] . Here we introduce a general method enabling a direct determination of the DW structure in ultrathin ferromagnets under ambient conditions. It relies on local measurements of the stray field distribution above the DW using a scanning nanomagnetometer based on the nitrogen-vacancy (NV) defect in diamond [16] , [17] , [18] . We first apply the method to a Ta/Co 40 Fe 40 B 20 (1 nm)/MgO magnetic wire and find clear signature of pure Bloch DWs. In contrast, we observe left-handed Néel DWs in a Pt/Co(0.6 nm)/AlO x wire, providing direct evidence for the presence of a sizable DMI in this multilayer stack. This method offers a new path for exploring interfacial DMI in ultrathin ferromagnets and elucidating the physics of DW motion under current. Principle of the method To convey the basic idea behind our method, we start by deriving analytical formulae of the magnetic field distribution at a distance d above a DW placed at x =0 in a perpendicularly magnetized film ( Fig. 1a ). The main contribution to the stray field, denoted by B ⊥ , is provided by the abrupt variation of the out-of-plane magnetization M z ( x )=− M s tanh( x / Δ DW ) (ref. 10 ), where M s is the saturation magnetization and Δ DW is the DW width parameter. 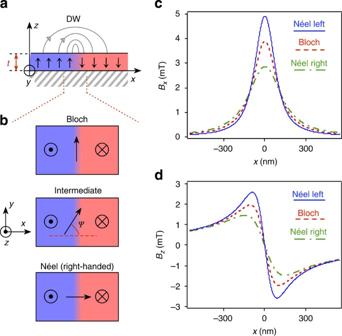Figure 1: Determining the nature of a DW by scanning nanomagnetometry. (a) Schematic side view of a DW in a perpendicularly magnetized film. The black arrows indicate the internal magnetization, while the grey arrows represent the magnetic field lines generated above the film. (b) Top view of the DW structure in a left-handed Bloch (top panel) or right-handed Néel (bottom panel) configuration, or an intermediate case characterized by the angleψ. (c,d) Calculated stray field components(c) and(d) at a distanced=120 nm above the magnetic layer, with a DW centred atx=0. Here we useMs=106A m−1andΔDW=20 nm. The resulting stray field components can be expressed as Figure 1: Determining the nature of a DW by scanning nanomagnetometry. ( a ) Schematic side view of a DW in a perpendicularly magnetized film. The black arrows indicate the internal magnetization, while the grey arrows represent the magnetic field lines generated above the film. ( b ) Top view of the DW structure in a left-handed Bloch (top panel) or right-handed Néel (bottom panel) configuration, or an intermediate case characterized by the angle ψ . ( c , d ) Calculated stray field components ( c ) and ( d ) at a distance d =120 nm above the magnetic layer, with a DW centred at x =0. Here we use M s =10 6 A m −1 and Δ D W =20 nm. Full size image where t is the film thickness. These approximate formulae are valid in the limit of (i) t ≪ d , (ii) Δ DW ≪ d and (iii) for an infinitely long DW along the y axis. On the other hand, the in-plane magnetization, with amplitude , can be oriented with an angle ψ with respect to the x axis ( Fig. 1b ). This angle is linked to the nature of the DW: ψ =± π /2 for a Bloch DW, whereas ψ =0 or π for a Néel DW. The two possible values define the chirality (right or left) of the DW. The spatial variation of the in-plane magnetization adds a contribution to the stray field, whose components are given by The net stray field above the DW is finally expressed as which indicates that a Néel DW (cos ψ =±1) produces an additional stray field owing to extra magnetic charges on each side of the wall. Using equations (1) and (2), we find a maximum relative difference in stray field between Bloch and Néel DWs scaling as ≈ π Δ DW /2 d . Local measurements of the stray field above a DW can therefore reveal its inner structure, characterized by the angle ψ . This is further illustrated in Fig. 1c,d , which shows the stray field components and for various DW configurations while using d =120 nm and Δ DW =20 nm, which are typical parameters of the experiments considered below on a Ta/CoFeB(1 nm)/MgO trilayer system. Magnetic field imaging with scanning-NV magnetometry We now demonstrate the effectiveness of the method by employing a single NV defect hosted in a diamond nanocrystal as a nanomagnetometer operating under ambient conditions [16] , [17] , [18] . Here the local magnetic field is evaluated within an atomic-size detection volume by monitoring the Zeeman shift of the NV defect electron spin sublevels through optical detection of the magnetic resonance. After grafting the diamond nanocrystal on the tip of an atomic force microscope (AFM), we obtain a scanning nanomagnetometer that provides quantitative maps of the stray field emanating from nanostructured samples [19] , [20] , [21] , with a magnetic field sensitivity in the range of 10 μT Hz −1/2 (ref. 22 ). In this study, the Zeeman frequency shift Δ f NV of the NV spin is measured while scanning the AFM tip in the tapping mode, so that the mean distance between the NV spin and the sample surface is kept constant with a typical tip oscillation amplitude of a few nanometres [20] . Each recorded value of Δ f NV is a function of and B NV, ⊥ , which are the parallel and perpendicular components, respectively, of the local magnetic field with respect to the NV spin’s quantization axis (see Supplementary Note 1 ). Note that a frequently found approximation is , where gμ B / h ≈28 GHz T −1 . This indicates that scanning-NV magnetometry essentially measures the projection of the magnetic field along the NV centre’s axis. The latter is characterized by spherical angles ( θ , φ ) measured independently in the ( xyz ) reference frame of the sample ( Fig. 2a ). 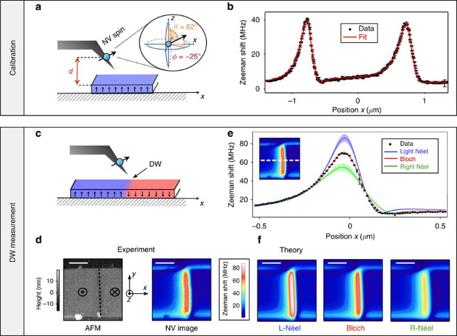Figure 2: Observation of Bloch DWs in a Ta/CoFeB/MgO wire. (a) The unknown parameters (distancedand productIs=Mst) are first calibrated by recording the stray field above a uniformly magnetized stripe. The inset defines the spherical angles (θ,ϕ) characterizing the NV spin’s quantization axis, measured independently. (b) Zeeman shift of the NV spin measured as a function ofx, across a 1.5-μm-wide stripe of Ta/CoFeB(1 nm)/MgO. The data (markers) are fitted to the theory (solid line), yieldingd=123±3 nm andIs=926±26 μA. (c) The stray field above a DW is then measured under the same conditions (same distanced, same NV spin). (d) AFM image (left panel) and corresponding Zeeman shift map (right panel) recorded on a 1.5-μm-wide stripe comprising a single DW. (e) Linecut across the DW (see dashed line in the inset). The markers are the experimental data, while the solid lines are the theoretical predictions for a Bloch (red), a left-handed Néel (blue) and a right-handed Néel DW (green). The shaded areas show 1 s.e. in the simulations due to uncertainties in the parameters (seeSupplementary Notes 3 and 5). (f) Theoretical two-dimensional Zeeman shift maps for the same three DW configurations. In bothe.f, the Bloch hypothesis is the one that best reproduces the data. Scale bar, 500 nm. Figure 2: Observation of Bloch DWs in a Ta/CoFeB/MgO wire. ( a ) The unknown parameters (distance d and product I s = M s t ) are first calibrated by recording the stray field above a uniformly magnetized stripe. The inset defines the spherical angles ( θ , ϕ ) characterizing the NV spin’s quantization axis, measured independently. ( b ) Zeeman shift of the NV spin measured as a function of x , across a 1.5-μm-wide stripe of Ta/CoFeB(1 nm)/MgO. The data (markers) are fitted to the theory (solid line), yielding d =123±3 nm and I s =926±26 μA. ( c ) The stray field above a DW is then measured under the same conditions (same distance d , same NV spin). ( d ) AFM image (left panel) and corresponding Zeeman shift map (right panel) recorded on a 1.5-μm-wide stripe comprising a single DW. ( e ) Linecut across the DW (see dashed line in the inset). The markers are the experimental data, while the solid lines are the theoretical predictions for a Bloch (red), a left-handed Néel (blue) and a right-handed Néel DW (green). The shaded areas show 1 s.e. in the simulations due to uncertainties in the parameters (see Supplementary Notes 3 and 5 ). ( f ) Theoretical two-dimensional Zeeman shift maps for the same three DW configurations. In both e . f , the Bloch hypothesis is the one that best reproduces the data. Scale bar, 500 nm. Full size image Calibration of the experiment We first applied our method to determine the structure of DWs in a 1.5-μm-wide magnetic wire made of a Ta(5 nm)/Co 40 Fe 40 B 20 (1 nm)/MgO(2 nm) trilayer stack (see Supplementary Note 2 ). This system has been intensively studied in the last years owing to low damping parameter and depinning field [23] . Before imaging a DW, it is first necessary to determine precisely (i) the distance d between the NV probe and the magnetic layer and (ii) the product I s = M s t , which are both directly involved in equation (3). These parameters are obtained by performing a calibration measurement above the edges of a uniformly magnetized wire, as shown in Fig. 2a . Here we use the fact that the stray field profile B edge ( x ) above an edge placed at x =0 can be easily expressed analytically in a form similar to equation (1), which only depends on d and I s . An example of a measurement obtained by scanning the magnetometer across a Ta/CoFeB/MgO stripe is shown in Fig. 2b . The data are fitted with a function corresponding to the Zeeman shift induced by the stray field B edge ( x )− B edge ( x + w c ), where w c is the width of the stripe (see Supplementary Note 3 ). Repeating this procedure for a set of independent calibration linecuts, we obtain d =123±3 nm and I s =926±26 μA, in good agreement with the value measured by other methods [24] . Bloch DW structure in a Ta/CoFeB/MgO wire Having determined all needed parameters, it is now possible to measure the stray field above a DW ( Fig. 2c ) and compare it with the theoretical prediction, which only depends on the angle ψ that characterizes the DW structure. To this end, an isolated DW was nucleated in a wire of the same Ta/CoFeB/MgO film and imaged with the scanning-NV magnetometer under the same conditions as for the calibration measurements. The resulting distribution of the Zeeman shift Δ f NV is shown in Fig. 2d together with the AFM image of the magnetic wire. Within the resolving power of our instrument, limited by the probe-to-sample distance d ~120 nm (ref. 20 ), the DW appears to be straight with a small tilt angle with respect to the long axis of the wire, determined to be 2±1°. Taking into account this DW spatial profile, the stray field above the DW was computed for (i) ψ =0 (right-handed Néel DW), (ii) ψ = π (left-handed Néel DW) and (iii) ψ ± π /2 (Bloch DW). Here we used the micromagnetic OOMMF software [25] , [26] rather than the analytical formula described above in order to avoid any approximation in the calculation (see Supplementary Note 4 ). The computed magnetic field distributions were finally converted into Zeeman shift distribution, taking into account the quantization axis of the NV spin. A linecut of the experimental data across the DW is shown in Fig. 2e , together with the predicted curves in the three above-mentioned cases. Excellent agreement is found if one assumes that the DW is purely of Bloch-type. The same conclusion can be drawn by directly comparing the full two-dimensional theoretical maps to the data ( Fig. 2d,f ). As described in detail in Supplementary Note 5 , all sources of uncertainty in the theoretical predictions were carefully analysed, yielding the 1-s.e. intervals shown as shaded areas in Fig. 2e . On the basis of this analysis, we find a 1-s.e. upper limit |cos ψ |<0.07. This corresponds to an upper limit for the DMI parameter D DMI , as defined in ref. 8 , of | D DMI |<0.01 mJ m −2 (see Supplementary Note 5 ). This result was confirmed on a second DW in the same wire. In addition, the measurements were reproduced for different projection axes of the NV probe. The results are shown in Fig. 3 for four NV defects with different quantization axes, showing excellent agreement between experiment and theory if one assumes a Bloch-type DW. These experiments provide an unambiguous confirmation of the Bloch nature of the DWs in our sample, but are also a striking illustration of the vector mapping capability offered by NV microscopy, allowing for robust tests of theoretical predictions. 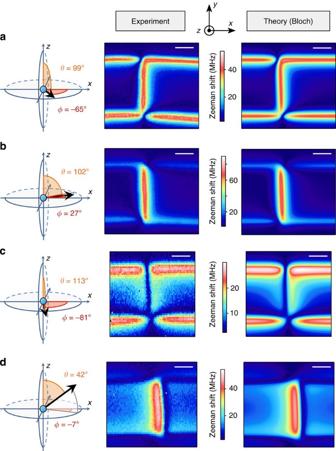Figure 3: Vector mapping of the DW stray field. Zeeman shift maps above a DW in a Ta/CoFeB/MgO wire recorded with different magnetometer’s projection axes (middle panels). The right panels show the corresponding calculated maps assuming a Bloch-type DW. The distancedis 116 nm (a), 122 nm (b), 195 nm (c) and 178 nm (d), respectively. The spherical angles (θ,ϕ) characterizing the projection axis are indicated on the left panels. Scale bar, 500 nm. Figure 3: Vector mapping of the DW stray field. Zeeman shift maps above a DW in a Ta/CoFeB/MgO wire recorded with different magnetometer’s projection axes (middle panels). The right panels show the corresponding calculated maps assuming a Bloch-type DW. The distance d is 116 nm ( a ), 122 nm ( b ), 195 nm ( c ) and 178 nm ( d ), respectively. The spherical angles ( θ , ϕ ) characterizing the projection axis are indicated on the left panels. Scale bar, 500 nm. Full size image We conclude that there is no evidence for the presence of a sizable interfacial DMI in a Ta(5 nm)/Co 40 Fe 40 B 20 (1 nm)/MgO trilayer stack. This is in contrast with recent experiments reported on similar samples with different compositions, such as Ta(5 nm)/Co 80 Fe 20 (0.6 nm)/MgO (refs 3 , 27 ) and Ta(0.5 nm)/Co 20 Fe 60 B 20 (1 nm)/MgO (refs 14 ), where a significant deviation towards Néel DWs was inferred from current-induced DW motion experiments. We note that contrary to these studies, our method indicates the nature of the DW at rest, in a direct manner, without any assumption on the DW dynamics. Our results therefore motivate a systematic study of the DW structure as a function of the composition of the trilayer stack. Left-handed Néel DW structure in a Pt/Co/AlO x wire In a second step, we explored another type of sample, namely a Pt(3 nm)/Co(0.6 nm)/AlO x (2 nm) trilayer grown by sputtering on a thermally oxidized silicon wafer (see Supplementary Note 2 ). The observation of current-induced DW motion with unexpectedly large velocities in this asymmetric stack has attracted considerable interest in the recent years [1] . Here the DW width is Δ DW ≈6 nm, leading to a relative field difference between Bloch and Néel cases of ≈8% at a distance d ≈120 nm. We followed a procedure similar to that described above. After a preliminary calibration of the experiment, a DW in a 500-nm-wide magnetic wire was imaged ( Fig. 4a,b ) and linecuts across the DW were compared with theoretical predictions ( Fig. 4c ). Here the experimental results clearly indicate a Néel-type DW structure with left-handed chirality. The same result was found for two other DWs. This provides direct evidence of a strong DMI at the Pt/Co interface, with a lower bound | D DMI |>0.1 mJ m −2 . This result is consistent with the conclusions of recent field-dependent DW nucleation experiments performed in similar films [28] . In addition, we note that the observed left-handed chirality, once combined with a damping-like torque induced by the spin-orbit terms, could explain the characteristics of DW motion under current in this sample [7] . 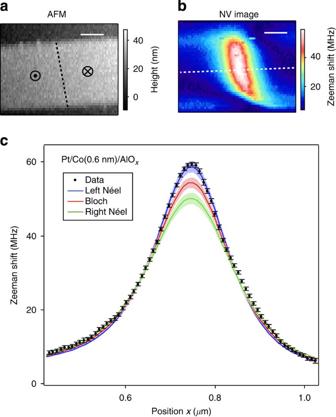Figure 4: Observation of left-handed Néel DWs in a Pt/Co/AlOxwire. (a) AFM image and (b) corresponding Zeeman shift map recorded by scanning the NV magnetometer above a DW in a 500-nm-wide magnetic wire of Pt/Co(0.6 nm)/AlOx. The spherical angles characterizing the NV defect quantization axis are (θ=87°,φ=23°). From calibration measurements above edges of the sample, we inferredd=119.0±3.4 nm andIs=671±18 μA (seeSupplementary Note 3). (c) Linecut extracted fromb(markers), together with the theoretical prediction (solid lines) for a Bloch (red), a left-handed Néel (blue) and a right-handed Néel DW (green). The shaded areas indicate 1 s.e. uncertainty in the simulations (seeSupplementary Note 5). Scale bar, 200 nm. Figure 4: Observation of left-handed Néel DWs in a Pt/Co/AlO x wire. ( a ) AFM image and ( b ) corresponding Zeeman shift map recorded by scanning the NV magnetometer above a DW in a 500-nm-wide magnetic wire of Pt/Co(0.6 nm)/AlO x . The spherical angles characterizing the NV defect quantization axis are ( θ =87°, φ =23°). From calibration measurements above edges of the sample, we inferred d =119.0±3.4 nm and I s =671±18 μA (see Supplementary Note 3 ). ( c ) Linecut extracted from b (markers), together with the theoretical prediction (solid lines) for a Bloch (red), a left-handed Néel (blue) and a right-handed Néel DW (green). The shaded areas indicate 1 s.e. uncertainty in the simulations (see Supplementary Note 5 ). Scale bar, 200 nm. Full size image In conclusion, we have shown how scanning-NV magnetometry enables direct discrimination between competing DW configurations in ultrathin ferromagnets. This method, which is not sensitive to possible artifacts linked to the DW dynamics, will help clarify the physics of DW motion under current, a necessary step towards the development of DW-based spintronic devices. In addition, this work opens a new avenue for studying the mechanisms at the origin of interfacial DMI in ultrathin ferromagnets, by measuring the DW structure while tuning the properties of the magnetic material [14] , [29] . This is a key milestone in the search for systems with large DMI that could sustain magnetic skyrmions [30] . How to cite this article: Tetienne, J.-P. et al. The nature of domain walls in ultrathin ferromagnets revealed by scanning nanomagnetometry. Nat. Commun. 6:6733 doi: 10.1038/ncomms7733 (2015).